A novel allosteric mechanism in the cysteine peptidase cathepsin K discovered by computational methods Allosteric modifiers have the potential to fine-tune enzyme activity. Therefore, targeting allosteric sites is gaining increasing recognition as a strategy in drug design. Here we report the use of computational methods for the discovery of the first small-molecule allosteric inhibitor of the collagenolytic cysteine peptidase cathepsin K, a major target for the treatment of osteoporosis. The molecule NSC13345 is identified by high-throughput docking of compound libraries to surface sites on the peptidase that are connected to the active site by an evolutionarily conserved network of residues (protein sector). The crystal structure of the complex shows that NSC13345 binds to a novel allosteric site on cathepsin K. The compound acts as a hyperbolic mixed modifier in the presence of a synthetic substrate, it completely inhibits collagen degradation and has good selectivity for cathepsin K over related enzymes. Altogether, these properties qualify our methodology and NSC13345 as promising candidates for allosteric drug design. Allostery is the coupling of conformational changes between two separated sites in proteins. In enzymes, one of the coupled positions is the active site and the other is the allosteric site. Binding of an effector at the allosteric site causes a conformational change, which results in modified enzyme activity. Therefore, targeting allosteric sites of enzymes is becoming increasingly popular as a strategy in drug development [1] , [2] , [3] , [4] . While targeting well-characterized allosteric sites is a straightforward task, allosteric drug design is more challenging when little or no data are available on this mode of regulation. Several methods have been successfully used for the identification of new allosteric sites, including high-throughput screening of compound libraries, phage display and tethering [5] . An alternative to these experimental approaches is posed by computational methods. One of the more popular and successful algorithms for investigating allosteric communication is the statistical coupling analysis (SCA), an evolution-based method that identifies conserved networks of residues in a protein family. Such networks have been termed protein sectors and represent the structural basis for allosteric communication [6] , [7] , [8] . The papain-like cysteine peptidase cathepsin K is being intensely studied due to its involvement in bone turnover, and a series of specific cathepsin K inhibitors have been developed for the treatment of osteoporosis. A detailed review of the biochemical properties, (patho)physiological roles and pharmacological targeting of cathepsin K has been published recently [9] . Cathepsin K is unique among human peptidases for its ability to cleave the triple helix of collagen molecules at multiple sites [10] , and its collagenolytic activity is modulated by glycosaminoglycans (GAGs) in a complex concentration-dependent manner [11] , [12] , [13] . The binding site for chondroitin sulphate is distant from the active site [14] and we have shown that sulphated GAGs act as allosteric regulators of cathepsin K [15] . Until now, this has remained the only experimentally characterized example of allosteric regulation in cysteine cathepsins. There have, however, been several other indications of allosteric regulation of cysteine cathepsins by GAGs and other polyanions. Heparin-like GAGs have been shown to affect the conformation and stability of cathepsin B as well as papain [16] , [17] , and a mechanism for the cathepsin B–heparin interaction has been proposed recently on the basis of computational results [18] . Moreover, heparan sulphate has been implicated in the regulation of the conformational plasticity of a cathepsin L homologue from Trypanosoma brucei , possibly by allosteric mechanisms [19] . Similarly, DNA has been shown to augment the inhibition of cathepsin V by serpins [20] . In this work, we combine SCA with computational surface site prediction and high-throughput docking to investigate allosteric regulation in the family of papain-like cysteine peptidases and to identify novel allosteric sites and modifiers of the model enzyme, cathepsin K. On the basis of these data, we identify and characterize the first reported small-molecule allosteric modifier of cathepsin K and a novel allosteric site on the enzyme, which is bound by this modifier. Furthermore, we investigate the functional importance of selected sector residues by alanine-scanning mutagenesis and characterize the effect of the identified inhibitor on one of these mutants. Altogether, the presented approach provides a novel alternative for allosteric drug design targeting papain-like cysteine peptidases and other enzymes. SCA of the papain-like cysteine peptidase family SCA was developed to identify networks of co-evolving residues in protein families and such networks have been proposed to mediate allosteric communication. In this work, we used SCA to analyse the family of papain-like cysteine peptidases, classified as peptidase subfamily C1A in the MEROPS database of peptidases [21] . We constructed a multiple-sequence alignment of 1,239 catalytic domains from this family. In most human cysteine cathepsins the catalytic domain accounts for the complete mature protein, in other species, however, it can be found as part of a larger protein architecture [21] . From the evolutionary perspective, residues within a protein can be divided into three groups: well-conserved residues, such as catalytic residues in the active site, co-evolving residues and residues that evolve independently from one another. First, we have identified well-conserved residues by calculating the positional conservation represented by the relative entropy D i for each position in the alignment ( Fig. 1a ). The cutoff value for well-conserved residues was arbitrarily set at D i >2 and these residues were mapped on the structure of cathepsin K (Protein Data Bank (PDB) accession code 1ATK ) ( Fig. 1b ). As expected, highest conservation energies were calculated for residues involved in catalysis (the positions of the catalytic diad Cys25 and His162 are marked), other residues in or near the active centre, three conserved disulphide bonds and several other residues (shown in detail in Supplementary Fig. 1 ). In the second step, the positional correlation matrix C i,j was calculated, which shows pairwise correlations between all pairs of positions in the alignment ( Fig. 1c ). To identify groups of co-evolving residues, the correlation matrix was clustered by hierarchical clustering ( Fig. 1d ). A detailed view of the clustered matrix together with the clustering dendrogram is shown in Supplementary Fig. 2 . Automated sector identification based on the calculated correlation values identified a single protein sector (boxed in Fig. 1d ), which was in agreement with the results obtained by manual examination of the clustering dendrogram (see Supplementary Fig. 2 ). Thorough examination of the clustered correlation matrix revealed further subdivision of sector residues, which is discussed in more detail in Supplementary Note 1 and Supplementary Fig. 3 . The spatial distribution of sector residues ( Fig. 1e ) shows a continuous network that surrounds the active site and stretches throughout the molecule. Comparison of positional conservation and pairwise coupling values showed that more than half of the residues identified as well conserved (20 out of 35) are also part of the protein sector. The remaining 15 residues comprise those that form the active centre, several conserved Gly residues and two conserved Ser and Pro residues (see Supplementary Fig. 1 for details). A complete representation of the protein sector together with conserved non-sector residues is shown in Fig. 1f . 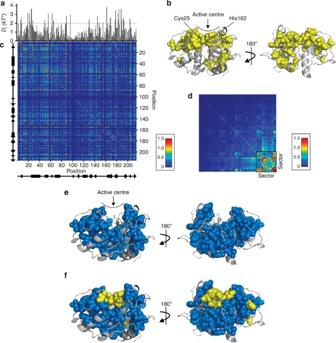Figure 1: Statistical coupling analysis of papain-like cysteine peptidases. (a) Positional conservationDiin the homologous superfamily. Residue positions correspond to mature human cathepsin K. The values ofDiare expressed in arbitrary energy units (kT*). (b) Well-conserved residues (relative entropyDi>2) mapped on the structure of cathepsin K in the front view (that is, the standard orientation, left panel) and in the back view of the molecule (right panel, rotated by 180° with respect to the left panel). Residues are shown as yellow spheres. (c) Positional correlation matrixCi,jin unclustered form. The matrix aligned with the graph in panel (a). Ribbon diagrams at the left and bottom sides of the matrix denote the distribution of secondary structure elements in the molecule. The colour scale varies linearly from 0kT*(blue) to 1.5kT*(red) (kT*is an arbitrary energy unit). (d) Correlation matrix clustered by hierarchical clustering. The portion that represents sector residues is boxed. The colour scale corresponds to panel (c). (e) Positions of sector residues in front view (left panel) and back view (right panel). Residues are shown as blue spheres. (f) Well-conserved and sector residues mapped together on cathepsin K. Residues are shown as spheres. The orientations and colour codes correspond to panels (b) and (e). Well-conserved residues that are also part of the sector are coloured blue. All molecular images were prepared using PyMOL (Schrödinger, Inc, Portland, OR, USA). Figure 1: Statistical coupling analysis of papain-like cysteine peptidases. ( a ) Positional conservation D i in the homologous superfamily. Residue positions correspond to mature human cathepsin K. The values of D i are expressed in arbitrary energy units ( kT* ). ( b ) Well-conserved residues (relative entropy D i >2) mapped on the structure of cathepsin K in the front view (that is, the standard orientation, left panel) and in the back view of the molecule (right panel, rotated by 180° with respect to the left panel). Residues are shown as yellow spheres. ( c ) Positional correlation matrix C i , j in unclustered form. The matrix aligned with the graph in panel ( a ). Ribbon diagrams at the left and bottom sides of the matrix denote the distribution of secondary structure elements in the molecule. The colour scale varies linearly from 0 kT* (blue) to 1.5 kT* (red) ( kT* is an arbitrary energy unit). ( d ) Correlation matrix clustered by hierarchical clustering. The portion that represents sector residues is boxed. The colour scale corresponds to panel ( c ). ( e ) Positions of sector residues in front view (left panel) and back view (right panel). Residues are shown as blue spheres. ( f ) Well-conserved and sector residues mapped together on cathepsin K. Residues are shown as spheres. The orientations and colour codes correspond to panels ( b ) and ( e ). Well-conserved residues that are also part of the sector are coloured blue. All molecular images were prepared using PyMOL (Schrödinger, Inc, Portland, OR, USA). Full size image The functional importance of sector residues in allosteric communication was analysed by alanine-scanning mutagenesis. Altogether, 15 single-substitution mutants were produced ( Supplementary Fig. 4 ). Most substitutions had a deleterious effect on the functionality of the mutant protein. Only one (mutant Pro50Ala) was obtained in active form and had activity similar to the wild type. More details are given in Supplementary Note 2 and Supplementary Figs 5,6 . Prediction of allosteric sites on cathepsin K Protein sectors have been proposed to mediate allosteric communication within proteins, it is thus expected that such networks will be directly connected to allosteric sites. Hence, allosteric sites can be predicted by identifying surface sites that are in direct contact with protein sectors. The validity of this assumption has been demonstrated for dihydrofolate reductase and PDZ domains [22] , [23] . Here we have used the AutoLigand [24] tool, which is part of the AutoDock Tools software package [25] , to predict binding cavities on the surface of cathepsin K ( Supplementary Fig. 7 ). A probe size of 50 points was chosen, which produces sufficiently large envelopes to accommodate the compounds used in the docking trials, that is, compounds with molecular masses between 150 and 500 Da, typically containing one or two cyclic systems and one or more functional groups. Filtering the predicted binding cavities according to the direct sector contact criterion identified eight potential allosteric sites as shown in Fig. 2 . As a validation of our hypothesis, one of these sites is the previously known chondroitin sulphate-binding site [14] , and the superposition of chondroitin sulphate from this complex (shown as sticks) onto the representation in Fig. 2 reveals multiple contacts with the protein sector. Apart from this site, seven other potential allosteric sites were predicted on the molecule. Of these, sites 2 and 3 contain relatively deep cavities, sites 1, 4, 6 and 7 form shallower clefts or pockets similar to the chondroitin sulphate-binding site and site 5 consists of an extended, relatively flat surface lined by several protruding loops. 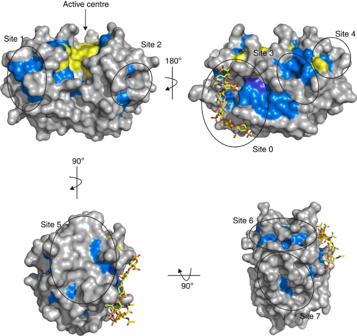Figure 2: Locations of the predicted allosteric sites on cathepsin K. Cathepsin K (PDB accession code1ATK) is shown in surface representation and is coloured according toFig. 1(well-conserved residues are yellow, sector residues are blue and the rest are grey). Chondroitin sulphate (from the cathepsin K/chondroitin sulphate complex, PDB accession code3C9E) was superposed onto this structure and is shown as sticks. The locations of seven potential allosteric sites on cathepsin K predicted by SCA and AutoLigand are marked by circles. All images were prepared using PyMOL (Schrödinger, Inc, Portland, OR, USA). As described in the following sections, site 6 was identified as a novel allosteric site in cathepsin K. Figure 2: Locations of the predicted allosteric sites on cathepsin K. Cathepsin K (PDB accession code 1ATK ) is shown in surface representation and is coloured according to Fig. 1 (well-conserved residues are yellow, sector residues are blue and the rest are grey). Chondroitin sulphate (from the cathepsin K/chondroitin sulphate complex, PDB accession code 3C9E ) was superposed onto this structure and is shown as sticks. The locations of seven potential allosteric sites on cathepsin K predicted by SCA and AutoLigand are marked by circles. All images were prepared using PyMOL (Schrödinger, Inc, Portland, OR, USA). Full size image Identification of compound 1 as an allosteric modifier To identify potential allosteric modifiers, diverse compound libraries from commercial vendors and non-profit organizations were retrieved from the ZINC database. The libraries were filtered to retain only molecules with molecular masses between 150 and 500 Da and six or less rotatable bonds. The filtered libraries were then docked to the seven predicted allosteric sites by a two-step docking procedure. In the first round, UCSF DOCK was used for high-throughput docking of the complete library. In the second round, top hits from the first round (top 10% of hits according to the values of the internal scoring function) were re-docked to the binding site with AutoDock [25] . Altogether, over 200 compounds targeting one or more of the predicted sites were selected for experimental verification and rigorously tested using synthetic substrates and collagen degradation assays. From these, 15 compounds had a measurable effect on cathepsin K activity in one or more assays. One of the most promising compounds was successfully characterized from both the structural and the functional perspectives and is presented in the following as a proof of concept. Compound 1 (2-[(2-carbamoylsulphanylacetyl)-amino]benzoic acid, NSC13345, chemical formula shown in Fig. 3a ) was identified from the NCI Diversity Set III compound library and was predicted to bind to sites 5 and 6 (see Fig. 2 ). For site 6, compound 1 was among the 0.5% top-scoring solutions from this library and for site 5 it ranked among the top 2%. Estimated equilibrium dissociation constants calculated by AutoDock (expressed by the program in terms of inhibition constants, K i ) were 170 μM for site 6 and 1.0 mM for site 5. The compound was experimentally confirmed as a modifier of cathepsin K and its characterization is described in detail in the next section. To identify the actual allosteric site, an inactive cathepsin K mutant (Cys25Ser) was crystallized in the presence of the compound. The complex crystallized in space group P 2 1 2 1 2 1 and the best crystal diffracted beyond 2.6 Å. The structure was solved by molecular replacement (diffraction and refinement statistics are collected in Table 1 ). The mutant contained eight propeptide residues at the N terminus, which remained after proenzyme processing with pepsin. Interestingly, this remnant binds to the active centre of the molecule in the adjacent crystal cell ( Supplementary Fig. 8 ). This interaction is, however, purely an artifact of crystallization and no indications of oligomer formation have been observed in solution neither on size-exclusion chromatography prior to crystallization nor in other experiments with this mutant that are outside of the scope of this manuscript. 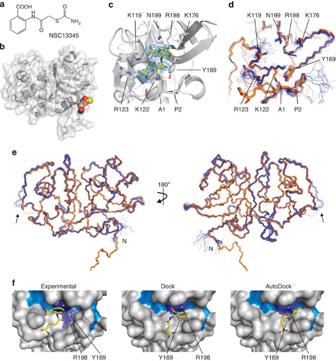Figure 3: Crystal structure of cathepsin K with bound compound1. (a) Chemical structure of compound1. (b) The location of the compound-1-binding site on cathepsin K. The enzyme is shown in the standard orientation in cartoon and solvent-accessible surface representation and the ligand is shown as spheres. (c) The electron density of the ligand in the maximum likelihood 2mFo–DFc map calculated with a ligand-free model and contoured at 1σ. Side chains of residues in close contact with compound1are shown as sticks and marked accordingly. (d) Superposition of cathepsin K with bound compound1(sticks) and an ensemble of all human cathepsin K structures available from the PDB (blue) at the compound-1-binding site. (e) Superposition of main chain atoms of cathepsin K with bound compound1(orange) and an ensemble of all human cathepsin K structures available from the PDB (blue). The region of conformational heterogeneity in the left subdomain is marked by an arrow. The flexible N terminus is marked by the letter ‘N’. (f) Comparison of the experimentally determined binding mode of compound1with the binding poses calculated by DOCK and AutoDock. The ligands are shown as sticks and the protein surface is coloured according toFig. 1(for clarity, sector residues are shown in alternating shades of blue). Sector residues in close contact with the ligand are indicated. Image in panelawas prepared using ChemDraw software (PerkinElmer Informatics, Inc., USA) and images in panelsb–fwere prepared using PyMOL (Schrödinger, Inc, Portland, OR, USA). Figure 3: Crystal structure of cathepsin K with bound compound 1 . ( a ) Chemical structure of compound 1 . ( b ) The location of the compound- 1 -binding site on cathepsin K. The enzyme is shown in the standard orientation in cartoon and solvent-accessible surface representation and the ligand is shown as spheres. ( c ) The electron density of the ligand in the maximum likelihood 2mFo–DFc map calculated with a ligand-free model and contoured at 1σ. Side chains of residues in close contact with compound 1 are shown as sticks and marked accordingly. ( d ) Superposition of cathepsin K with bound compound 1 (sticks) and an ensemble of all human cathepsin K structures available from the PDB (blue) at the compound- 1 -binding site. ( e ) Superposition of main chain atoms of cathepsin K with bound compound 1 (orange) and an ensemble of all human cathepsin K structures available from the PDB (blue). The region of conformational heterogeneity in the left subdomain is marked by an arrow. The flexible N terminus is marked by the letter ‘N’. ( f ) Comparison of the experimentally determined binding mode of compound 1 with the binding poses calculated by DOCK and AutoDock. The ligands are shown as sticks and the protein surface is coloured according to Fig. 1 (for clarity, sector residues are shown in alternating shades of blue). Sector residues in close contact with the ligand are indicated. Image in panel a was prepared using ChemDraw software (PerkinElmer Informatics, Inc., USA) and images in panels b – f were prepared using PyMOL (Schrödinger, Inc, Portland, OR, USA). Full size image Table 1 X-ray data collection and refinement statistics. Full size table Compound 1 was identified bound at the lower right side of cathepsin K ( Fig. 3b ). The binding site corresponds to site 6 in Fig. 2 and was thereby identified as a novel allosteric site in cathepsin K. The electron density of compound 1 was well visible in the maximum likelihood 2mFo–DFc map calculated with a ligand-free model ( Fig. 3c ). A stereo image of the electron density in this part of the structure is shown in Supplementary Fig. 9 . In the structure, compound 1 forms close contacts with at least eight residues of the receptor (shown as sticks and marked in Fig. 3c ). The complete list of close contacts observed in the crystal structure is provided in Supplementary Table 1 . To investigate putative conformational changes induced in the protein on ligand binding, we have superposed the cathepsin K/compound 1 complex and all other structures of human cathepsin K currently available from the worldwide PDB. The relatively large number of available crystal structures (counting a total of 36 structures, accession codes are collected in Supplementary Table 2 ) provides sufficient information for reasonably good insight into the conformational space of the protein. As shown in Fig. 3d (the reported crystal structure is shown as sticks and all other structures are shown as lines), the binding site has a dynamic shape due to the flexible N terminus of the mature protein (involving mostly residues Ala1 and Pro2) and flexible side chains of Lys119 and Arg123. Altogether, only the side chain of Lys122 undergoes a significant conformational change on binding of compound 1 , while all other residues adopt conformations that do not deviate significantly from the conformational space of ligand-free cathepsin K. Similarly, no major deviations in the positions of backbone atoms were observed in the complex in comparison with other available structures ( Fig. 3e ). From this figure, it is also worth noting a conformational heterogeneity in the left subdomain of the molecule that involves residues Met97 through Thr101 or in one case Met97 through Ala104 (marked by an arrow) and was to the best our knowledge not observed before. Regardless of the apparent lack of a conformational change, the shape of the binding site changed significantly on ligand binding in comparison with the structure of the receptor used in the docking trials (PDB accession code 1ATK ). Therefore, the actual binding mode of compound 1 differs from the calculated poses where a rigid-body model of the receptor was used ( Fig. 3f ). Nevertheless, both programs correctly identified not only the binding of the compound at this site but also most residues in close contact with the ligand, including both sector residues (Arg198 and Tyr169). Properties of compound 1 as a modifier The properties of compound 1 as a modifier of cathepsin K activity were tested in three independent assays, one using a low-molecular-mass synthetic fluorescent substrate and two assays using macromolecular substrates. The compound had very little effect on the hydrolysis of Z–FR–AMC, the synthetic substrate routinely used for measuring cathepsin K activity. Its kinetic profile was therefore characterized using the internally quenched substrate Abz–HPGGPQ–EDDnp that, in contrast to Z–FR–AMC, binds along the whole active centre of the enzyme. While the effect of compound 1 on the hydrolysis of this substrate is still small, it is nonetheless sufficient for the characterization of its action. The kinetic mechanism was diagnosed by the specific velocity plot [26] where initial reaction rates are measured at varying substrate and inhibitor concentrations and then plotted as shown in Fig. 4a . This method allowed for an unambiguous identification of compound 1 as a hyperbolic mixed modifier with predominantly competitive character. Although cooperativity can occur in monomeric enzymes [27] , allosteric interactions in cathepsin K ensue in the absence of cooperativity as in many other systems [28] . Hyperbolic mixed modification is the fundamental mechanism of allosteric interactions, which occurs in different variants of the general modifier mechanism [29] . To determine the kinetic parameters, additional kinetic experiments were performed and are presented in Fig. 4b in a plot of residual enzyme activity versus modifier concentration. From the combination of these experiments the kinetic parameters were calculated as K i =28±8 μM, α =2.4±0.4 and β =1.3±0.2 for the interaction of compound 1 with cathepsin K. The value of α >1 indicates decreased affinity of the enzyme for the substrate when the modifier is bound, while the value of β >1 signifies a concomitant increase in the catalytic rate of the enzyme. This particular combination represents a mechanism in which the modifier behaves as inhibitor below a critical substrate concentration that, in terms of the [S]/ K m ratio σ , can be defined as σ 0 =( β – α )/(1– β ). Above σ 0 the modifier behaves as an activator, while no effects at all can be measured if σ = σ 0 . Since for this system σ 0 =3.7, performing experiments at [S]≈4 × K m or higher would be experimentally difficult due to the inner filter effect of the substrate and would result in reaction rates hardly distinguishable from controls. In any case, the value of β is close to 1 and this kinetic behaviour is thus similar to that of a hyperbolic competitive inhibitor that acts purely by reducing the affinity of the enzyme for the substrate without affecting the catalytic rate. This kinetic mechanism, in which the modifier behaves as either an inhibitor or an activator, is rare but has been documented in a few cases, for example, in butyrylcholinesterase [30] . 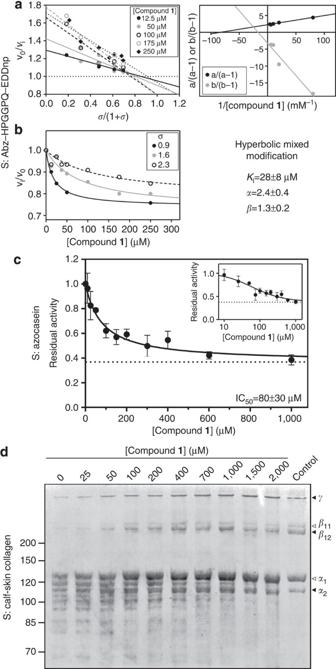Figure 4: Characterization of the inhibitory properties of compound1. (a) The kinetic mechanism of compound1analysed by the specific velocity plot. Experiments were performed using the synthetic substrate Abz–HPGGPQ–EDDnp. The primary specific velocity plot is shown in the left panel and the replot is shown in the right panel.σ=[S]/Km. (b) The plot of residual enzyme activity as a function of inhibitor concentration together with the interaction parameters calculated from the combination of experiments in panels (a) and (b). Experiments were performed using the synthetic substrate Abz–HPGGPQ–EDDnp.σ=[S]/Km, and the coefficientsαandβare derived from equation (2) and determine the inhibition mechanism. (c) Effect of compound1on azocasein degradation by cathepsin K. Error bars represent the s.e.m. of three experiments. Equation (5) was fitted to the experimental data and used to determine the IC50value. The inset shows the same data plotted on a semi-logarithmic scale. (d) Effect of compound1on the collagenolytic activity of cathepsin K followed by SDS–PAGE. All experiments were performed in 100 mM sodium acetate buffer, pH 5.5, containing 1 mM EDTA and 2.5 mM DTT, as described in detail in the Methods section. The plots were created with GraphPad Prism 5.0 (GraphPad Software, La Jolla, CA, USA). Figure 4: Characterization of the inhibitory properties of compound 1 . ( a ) The kinetic mechanism of compound 1 analysed by the specific velocity plot. Experiments were performed using the synthetic substrate Abz–HPGGPQ–EDDnp. The primary specific velocity plot is shown in the left panel and the replot is shown in the right panel. σ =[S]/ K m . ( b ) The plot of residual enzyme activity as a function of inhibitor concentration together with the interaction parameters calculated from the combination of experiments in panels ( a ) and ( b ). Experiments were performed using the synthetic substrate Abz–HPGGPQ–EDDnp. σ =[S]/ K m , and the coefficients α and β are derived from equation (2) and determine the inhibition mechanism. ( c ) Effect of compound 1 on azocasein degradation by cathepsin K. Error bars represent the s.e.m. of three experiments. Equation (5) was fitted to the experimental data and used to determine the IC 50 value. The inset shows the same data plotted on a semi-logarithmic scale. ( d ) Effect of compound 1 on the collagenolytic activity of cathepsin K followed by SDS–PAGE. All experiments were performed in 100 mM sodium acetate buffer, pH 5.5, containing 1 mM EDTA and 2.5 mM DTT, as described in detail in the Methods section. The plots were created with GraphPad Prism 5.0 (GraphPad Software, La Jolla, CA, USA). Full size image Studying the effect of modifiers on the hydrolysis of a synthetic substrate is practical because it allows for easy determination of the kinetic mechanism and calculation of the binding constant. However, these results must not be generalized and a priori held true for macromolecular substrates. Therefore, we have tested the effect of compound 1 on the hydrolysis of two protein substrates: calf-skin collagen, which is composed mostly of type I collagen, the major natural substrate of cathepsin K, and azo dye-labelled casein as a non-specific protein substrate. The effect of compound 1 on the hydrolysis of azocasein was similar to that obtained with the synthetic substrate ( Fig. 4c ). The compound behaved as a hyperbolic inhibitor reducing the hydrolytic rate to about 40% of the initial rate with an IC 50 value of 80±30 μM. The collagenolytic activity was tested semi-qualitatively by following the fragmentation of the characteristic type I collagen pattern into smaller products on SDS–PAGE after incubation of the samples with cathepsin K in the presence of increasing concentrations of compound 1 ( Fig. 4d ). Unlike the behaviour in presence of the synthetic substrate and azocasein, compound 1 completely inhibited the collagenolytic activity of cathepsin K and the IC 50 value was estimated at about 100–200 μM. The relationship between IC 50 and K i depends on the kinetic parameters α , β and K m as well as [S]. In general, IC 50 is a bad estimator of K i (ref. 31 ). IC 50 and K i are interconvertible when the kinetic mechanism is well characterized. However, using ill-defined macromolecular substrates such as azocasein and collagen makes such a comparison impossible because individual kinetic parameters cannot be determined. Also, changing the substrate can change the kinetic mechanism, which is the case of the cathepsin K–collagen–compound 1 system because β =0 with collagen as substrate and the kinetic mechanism of inhibition becomes linear mixed ( α >1 and β =0). Nonetheless, we can readily compare the IC 50 values between all experiments by reanalyzing the data obtained with the synthetic substrate ( Fig. 4b ) with equation (5). The obtained IC 50 values of 80±30 and 120±30 μM for σ =1.6 and σ =2.3, respectively, are directly comparable to the IC 50 values calculated in macromolecular assays. Interaction of compound 1 with other cysteine peptidases To determine the selectivity of compound 1 we have evaluated its inhibitory activity against other cysteine peptidases, including human cathepsins L, S and V that are closely related to cathepsin K as well as human cathepsin B, a ubiquitous and widely studied cysteine cathepsin [32] , and papain as the archetypal representative of the family. The azocasein assay was used for the comparison, because this substrate is effectively cleaved by all tested peptidases. Compound 1 reduced the activity of cathepsins L, S, V and B in a concentration-dependent manner ( Supplementary Fig. 10 ), whereas only a minor reduction of papain activity was observed (about 5% at the highest substrate concentration). The IC 50 values collected in Table 2 show that compound 1 has at least 20-fold selectivity for cathepsin K over other cysteine cathepsins. Due to the limited solubility of compound 1 (up to about 3 mM under the conditions used in these experiments), residual enzyme activity at saturation with compound 1 could not be determined for these enzymes. Table 2 Effect of compound 1 on the activity of different cysteine cathepsins. Full size table Whether these off-target effects are mediated via the same allosteric mechanism or by other specific or non-specific means remains to be determined. Docking experiments in silico supported the experimental findings by showing that the binding of compound 1 at the analogous sites in other cathepsins would be considerably less favourable than in cathepsin K ( Supplementary Fig. 11 ). Active site-directed probes for peptidases have been intensively studied in the past decades [33] , and cathepsin K inhibitors, such as odanacatib, are showing promising results in clinical trials for the treatment of osteoporosis [34] . In this paper we describe the first low-molecular-weight allosteric modifier of cathepsin K. Compared with active site-directed inhibitors, which essentially act as an on/off switch, allosteric modifiers can be designed to fine-tune enzyme activity and thereby circumvent some of the adverse effects of active site-directed inhibitors, such as over-potency and interference with off-target biological functions. Compound 1 has all the characteristics theoretically expected from allosteric modifiers, but rarely observed in practice. The compound can completely abolish collagen degradation, which is the target in the treatment of osteoporosis, while only partially inhibiting the activity on off-target substrates, exemplified here by a synthetic fluorescent probe and a non-specific protein substrate (azocasein). Compound 1 also has good selectivity for cathepsin K over other related enzymes and thus provides a solid basis for the design of drugs for the treatment of patients with osteoporosis. At the molecular level, kinetic and structural data are in agreement that binding of compound 1 causes no significant conformational changes in cathepsin K. Instead, the allosteric effect is likely mediated by alterations in protein dynamics or population shifts within the usual conformational space of the enzyme. Such effects have been described previously, for example, for the binding of cyclic AMP to cyclic-AMP-binding protein [35] , and are reviewed in detail in Tsai et al. [36] In the case of cathepsin K these effects are only able to reduce the rates of hydrolysis for small, easily hydrolysable substrates by a limited extent, however, in the case of the bulky triple helix of collagen they are sufficient to completely inhibit its degradation. Similar to compound 1 , the binding of chondroitin-4-sulphate, an allosteric activator of cathepsin K [15] , caused no apparent conformational changes in the molecule [14] . It is also worth noting that no crystal structure of cathepsin K with a vacant active centre is available to-date, as each of the available structures contains a bound inhibitor molecule in the active centre, which is in our case substituted by the propeptide of the crystal neighbour, as discussed above. Therefore, a direct comparison with a truly ligand-free cathepsin K molecule cannot be made. The primary premise of this work was that allosteric sites can be predicted by computational means. The combination of SCA to identify networks that transmit allosteric signals within the protein and AutoLigand to predict binding sites on the protein surface proved successful. In addition to compound 1 , several other probes have been identified and are currently under investigation. The site identified in this study is the third known allosteric site on cathepsin K next to the chondroitin sulphate-binding site [14] and to a site corresponding to site 7 in Fig. 2 that has been predicted on the bottom of the molecule as a second binding site for heparin [15] . It remains to be determined whether the novel allosteric site is used by a natural effector or represents an orphan site. Interestingly, a recent computational study predicted that heparin regulates cathepsin B stability by binding to the site analogous to the compound- 1 -binding site [18] . Altogether these data demonstrate that allosteric regulation is a common mechanism in papain-like peptidase regulation, despite the scarce availability of experimental data. In addition to the presented results, we have also observed conformational heterogeneity from the superposition of all available cathepsin K structures ( Fig. 3e ), which has to our knowledge remained undetected until now. The involved loop (residues Met97 through Thr101) lines the binding pocket designated as site 4 in Fig. 2 and its flexibility may indicate the existence of a further allosteric site in cathepsin K. SCA has been used previously to investigate allosteric communication in several different protein families, including small model proteins, such as the PDZ and WW domains [37] , [38] , as well as larger proteins, such as G proteins [39] , [40] , Hsp70 chaperones [41] and TonB-dependent transporters [42] . The most relevant comparison with papain-like cysteine peptidases is the analysis of the functionally similar S1 family of chymotrypsin-like serine peptidases [7] , [8] . In this family, three independent protein sectors were identified, whereas the papain family contains only one sector. All three sectors in chymotrypsin were functionally characterized by alanine-scanning mutagenesis and were found to be responsible for different properties of the enzyme, such as thermal stability and catalytic properties [8] . In cathepsin K, most sector mutations proved deleterious. While the deleterious effect of replacing bulky aromatic residues (for example, five mutants replaced a Tyr residue by Ala) can be in part explained by their immutability, these results also indicate that a fully functional sector is necessary for a functional peptidase. This complies with a recent study showing that sector positions in PDZ domains are functionally more sensitive to mutation than non-sector residues [37] . Moreover, the destructive effects of naturally occurring mutations in the CATK gene have been described in patients suffering from the rare genetic disease pycnodysostosis [9] . Importantly, compound 1 has been shown to be an effective allosteric inhibitor of cathepsin K with limited effect on other related enzymes and is thus an attractive candidate for drug design and a valuable probe for studying the mechanisms of cathepsin K function. Materials All recombinant human cysteine cathepsins, including wild types and mutants, were produced in Escherichia coli by the protocol described previously [43] . All substitution mutants were prepared using the Agilent QuikChange II Site-Directed Mutagenesis Kit (Santa Clara, CA, USA) according to the manufacturer’s instructions. Papain was purchased from Sigma-Aldrich (St Louis, MO, USA). All active enzyme concentrations were determined by active site titrations using the irreversible inhibitor E-64 (Bachem, Bubendorf, Switzerland). Compound 1 (2-[(2-carbamoylsulphanylacetyl)-amino]benzoic acid) was obtained from the US NCI/DTP Open Chemical Repository (compound ID NSC 13345). Multiple-sequence alignment Sequences of proteins from the C1A subfamily of peptidases were retrieved from the MEROPS database [21] . Coordinates for all known structures of proteins from the C1A peptidase family (papain-like fold) were obtained from the PDB. These coordinates were used to construct a structure-based sequence alignment of these proteins using the UCSF Chimera software package [44] , which served as a basis for manual refinement of the final alignment. Statistical coupling analysis The SCA was performed in the MATLAB environment (The MathWorks, Inc., Natick, MA, USA) using versions 4 and 5 of the SCA software package. All calculations were performed according to the packages’ documentation, which also contains a detailed description of the theoretical principles underlying SCA [45] . Prior to the analysis the alignment was truncated to the sequence of human cathepsin K, which was used throughout the analysis to visualize the results and filtered to retain only sequences with a maximal pairwise sequence identity of 80% to remove statistical bias. Binding-site identification Potential ligand-binding sites on the surface of cathepsin K (PDB accession code 1ATK ) were predicted using AutoLigand [24] , which is part of the AutoDock Tools software package [25] . The calculations were performed using a probe of 50 dots. A total of 30 solutions were calculated and ranked according to the energy per volume score of the internal scoring function. Docking of compound libraries Compound libraries were obtained from the ZINC database [46] . Specifically, the compound identified in this study was from the NCI Diversity 3 dataset, which contains 1,597 compounds. Other libraries used were the Aldrich CPR dataset (over 180,000 compounds), Sigma-Aldrich Building Blocks dataset (over 60,000 compounds), the Acros Organics dataset (over 15,000 compounds), the ChemBridge Building Blocks dataset (over 14,000 compounds) and the Bachem dataset (over 4,000 compounds). The libraries were pre-filtered to retain only molecules with molecular masses between 150 and 500 Da and molecules containing more than six rotatable bonds were discarded to reduce the effect of entropic change on binding. Docking of compound libraries was performed with DOCK 6.4 (UCSF, CA, USA). Each binding site was defined manually according to the instructions included with the DOCK 6.4 program suite (available online at http://dock.compbio.ucsf.edu/ ). The best hits (about top 10%) were selected on the basis of the binding energies calculated by the internal scoring function and re-docked to the receptor using AutoDock [25] . The best binders were again selected on the basis of their binding affinities calculated by the AutoDock internal scoring function. Each binding site on the receptor (cathepsin K, PDB accession code 1ATK ) was first defined manually and the grid calculated with AutoGrid 4.2. Each ligand was parameterized to allow the maximum number of rotatable bonds, but excluding amide and ring bonds. Docking was performed with the Lamarckian genetic algorithm. For each ligand, 20 runs were performed using a population of 300 individuals over 3,000 generations, starting from random orientations and conformations. Kinetic measurements All kinetic measurements were performed in 100 mM sodium acetate buffer, pH 5.5, containing 1 mM EDTA and 2.5 mM dithiothreitol (DTT) in single-use acrylic cuvettes (1 × 1 cm) thermostatted at 25±1 °C with magnetic stirring. Hydrolysis of the internally quenched substrate Abz–HPGGPQ–EDDnp (Merck Millipore, Darmstadt, Germany) was followed fluorometrically at λ ex =320 nm and λ em =420 nm. Hydrolysis of Z–FR–AMC was followed fluorometrically at λ ex =383 nm and λ em =455 nm. Both substrate and compound 1 were analysed spectroscopically to determine their absorption properties under assay conditions and appropriate corrections were made to the calculated reaction rates to take into account the inner filter effect [47] . The K m values for the quenched substrate were 3.8±0.5 and 2.7±0.3 μM for wild-type cathepsin K and mutant Pro50Ala, respectively, and the k cat values were 2.9±0.1 s −1 and 2.0±0.1 s −1 , respectively. Collagenolytic assay Soluble calf-skin collagen (Worthington Biochemical Corporation, Lakewood, NJ, USA) was diluted in 100 mM sodium acetate buffer, pH 5.5, containing 1 mM EDTA and 5 mM DTT to a final concentration of 0.5 mg ml −1 . Experiments were started by addition of cathepsin K (wild-type or mutant Pro50Ala, final enzyme concentration 0.5 μM) to the reaction mixture containing collagen and modifier (final concentration 1 mM or lower, depending on the solubility). All assays were performed at 25±1 °C with shaking on an Eppendorf Thermomixer Comfort. Samples were incubated for 2 hours and the reaction was blocked by addition of E-64 to a final concentration of 1 μM. Ten micrograms of digested collagen were analysed by SDS–PAGE on 8% polyacrylamide gels and protein bands were stained with Coomassie Brilliant Blue R-250. Azocasein degradation assay Azocasein (Sigma-Aldrich, USA) was dissolved in 100 mM sodium acetate buffer, pH 5.5, containing 1 mM EDTA and 5 mM DTT at a concentration of 3 mg ml −1 . The samples were incubated for 30 minutes at 37 °C with 0.5 μM enzyme (cathepsin K, L, S, B, V or papain) in the presence of increasing concentrations of compound 1 . Reactions were stopped by addition of trichloroacetic acid (final concentration 5% v/v), centrifuged, clear supernatants mixed with 0.5 M NaOH and the concentrations of solubilized peptides determined by A 440 measurements. Appropriate blanks were run to take into account the absorption of azocasein and compound 1 alone. Kinetic models The effect of compound 1 on enzymatic activity was analysed with the general modifier mechanism [48] . Assuming quasi-equilibrium conditions, K S ≈ K m , the reaction rate is defined by equation (1): where v 0 is the reaction rate in the absence of modifier, K i is the inhibition constant, α and β are dimensionless coefficients and σ =[S]/ K m . To determine the mechanism of interaction, plot the kinetic data and calculate preliminary values of the interaction parameters, the specific velocity plot was used [26] . For this purpose, equation(1) is rewritten as: The plot of v 0 / v i versus σ /(1+ σ ) produces straight lines with intersection points at v 0 / v i =1, regardless of the interaction mechanism. The parameters α , β and K i are determined by replotting the extrapolated values of the straight lines at σ /(1+ σ )=0 (a) and σ /(1+ σ )=1 (b) versus 1/[I] in the form: The effect of compound 1 on azocasein degradation was analysed using a modified form of the four-parameter logistic equation adapted to enzyme inhibition considering the Hill coefficient h =1: where v ∞ is the residual reaction rate at saturation with inhibitor and IC 50 is the inhibitor concentration necessary to achieve a half-maximal effect, that is, midway between v 0 and v ∞ . The value of IC 50 is used here as an empirical comparison term for assessing inhibitor efficiency towards different enzymes using an ill-defined substrate. It should not be confused with the concentration of inhibitor necessary to reduce enzyme activity to one half of its value in the absence of modifier. All mathematical analyses and graphical manipulations were performed with GraphPad Prism 5.0 (GraphPad Software, La Jolla, CA, USA). Crystallization and structure determination Procathepsin K Cys25Ser was produced in E. coli and purified as described previously [43] . To remove the propeptide, the proenzyme was processed with pepsin (final concentration 20 μg ml −1 ) for 1 h at 37 °C in 100 mM sodium acetate buffer, pH 4.0, containing 500 mM NaCl. The processed catalytic domain was separated from other components by size-exclusion chromatography on a Superdex 75 column (GE Healthcare, USA), dialyzed against 100 mM sodium acetate buffer, pH 4.0, containing 500 mM NaCl and concentrated to the maximum achievable concentration (5 mg ml −1 of soluble protein). Crystals were grown by the sitting drop vapour diffusion method at 20 °C for ~14 days. The reservoir contained 200 μl of 0.2 M ammonium sulphate, pH 5.5, 30% (w/v) PEG-8000 and the drop was composed of 1 μl of reservoir solution containing 5 mM compound 1 and 1 μl of the protein solution. Prior to data collection, the crystal was immersed in a cryoprotective solution containing 0.2 M ammonium sulphate, pH 5.5, 30% (w/v) PEG-8000 and 25% (v/v) glycerol. Diffraction data were collected from a single crystal at 100 K on a Bruker X8 Proteum diffractometer equipped with a rotating Cu anode (wavelength of emitted X-rays of 1.54 Å) and a Platinum 135 CCD detector. The collected data were processed and scaled with the accompanying PROTEUM2 software. The diffraction data and refinement statistics are collected in Table 1 . The orientation and position of the protein were determined by molecular replacement using the Phaser module in the Phenix software suite (version 1.8.2). The crystal structure of wild-type human cathepsin K (PDB accession code 1ATK ) was used as the search model. Model building was performed using Coot software [49] (version 0.7) and the phenix.refine module was used for electron density modification and refinement. Accession codes: The coordinates and structure form factors of human cathepsin K in complex with compound 1 were deposited in the RCSB Protein Data Bank under accession code 4LEG . These data can be obtained via http://www.rcsb.org/pdb/home/home.do . How to cite this article: Novinec, M. et al. A novel allosteric mechanism in the cysteine peptidase cathepsin K discovered by computational methods. Nat. Commun. 5:3287 doi: 10.1038/ncomms4287 (2014).